Activation of G-protein-coupled receptors correlates with the formation of a continuous internal water pathway Recent crystal structures of G-protein-coupled receptors (GPCRs) have revealed ordered internal water molecules, raising questions about the functional role of those waters for receptor activation that could not be answered by the static structures. Here, we used molecular dynamics simulations to monitor—at atomic and high temporal resolution—conformational changes of central importance for the activation of three prototypical GPCRs with known crystal structures: the adenosine A 2A receptor, the β 2 -adrenergic receptor and rhodopsin. Our simulations reveal that a hydrophobic layer of amino acid residues next to the characteristic NPxxY motif forms a gate that opens to form a continuous water channel only upon receptor activation. The highly conserved tyrosine residue Y 7.53 undergoes transitions between three distinct conformations representative of inactive, G-protein activated and GPCR metastates. Additional analysis of the available GPCR crystal structures reveals general principles governing the functional roles of internal waters in GPCRs. Internal water molecules are essential for the function of many membrane proteins such as channel and transport proteins [1] . For G-protein-coupled receptors (GPCRs), which form the largest class of membrane proteins transmitting extracellular signals across the plasma membrane, internal water molecules have been proposed to play an important role for receptor activation but mechanistic models remain speculative [2] . Previous studies revealed that water molecules from the cytoplasmic region of rhodopsin (Rho) are involved in the hydrolytic release of retinal upon Rho activation by light [3] , [4] . Crystal structures of Rho and the beta-2 adrenergic receptor (β 2 AR) revealed further details. Distinct conformational changes occur during activation of these receptors, including reorganizations of inner protein hydrogen bonding networks, which could be in contact with internal waters [5] , [6] . An important step forward came from the recent high-resolution crystal structures of the A 2A adenosine receptor (A 2A R) and the delta opioid receptor (δOR), which revealed internal ordered water molecules that could be crucial for GPCR activation [7] , [8] . On the basis of their crystal structures, Liu et al. [7] proposed that the A 2A R in the non-activated state contains a nearly continuous internal water channel, which is disrupted in the activated receptor. However, this detailed suggestion on the extension of the internal water channel is not conclusive for several reasons: (1) As is shown in this article, the A 2A receptor’s internal water molecules are quite mobile, which exclude determination of their precise spatial localization within the protein’s structural framework. (2) To calculate the receptor’s intrinsic water pathway, Liu et al. [7] increased the radius of water molecules and connected all water molecules with each other because it is not possible to distinguish between a continuous and a discontinuous water channel from crystal structures. However, it is important to know the exact spatiotemporal distribution of water inside of GPCRs and their contact sites with the receptor’s polypeptide backbone and side chains to finally understand the relationship of an internal water channel to the receptor’s function. Internal waters can strongly interfere with internal hydrogen bonding networks of a protein’s backbone and side chains, thereby strongly influencing its conformational and structural changes. Notably, the details of how the intrinsic water molecules couple to the protein structure and thereby affect GPCR activation at the atomic level cannot be solved by static X-ray structures. Alternatively, molecular dynamics (MD) simulations can resolve atomic details of structural transitions of receptors and their internal waters, which are experimentally not accessible [8] , [9] , [10] , [11] . Here, by using a total of 32-μs all-atom MD simulations, we studied with high spatial and temporal resolution important steps during the activation of three different receptors from class A GPCRs to elucidate how water molecules enter the inner space of a receptor, couple to and influence this protein’s structural transitions. Contrary to Liu et al. [7] , our simulations revealed that in the inactivated state of the A 2A R the internal water pathway is interrupted by a gate of hydrophobic amino acids, which upon receptor activation evoke conformational changes opening a continuous internal water channel. By analyzing all presently available GPCR crystal structures we were able to identify common functional roles of internal waters within the members of class A GPCRs. Hydrophobic layers of amino acid residues in the A 2A R We started our MD investigations from the 1.8-Å resolution A 2A R (PDB 4EIY) crystal structure [7] , which shows a comprehensive network of 57 solvent molecules inside the receptor together with a sodium ion at the allosteric site. According to the crystallographic b-factors ( Fig. 1a ) many of the receptor’s intrinsic water molecules are mobile, a property further manifested by the poor electron density map in several regions of the receptor, especially those close to Y288 7.53 in the NPxxY motif and D52 2.50 at the allosteric site. Meanwhile, another 1.8-Å resolution GPCR crystal structure, that of the DOR (PDB 4N6H), was released [12] . This also contains internal waters just as the A 2A R does ( Fig. 1b ). 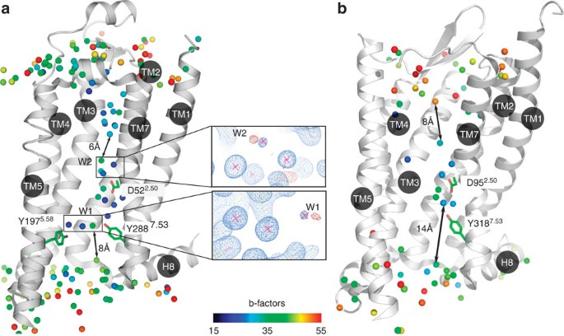Figure 1: Water molecules and hydrophobic layers of amino acid residues in the crystal structures of adrenergic and opioid receptors. (a) A2AR (PDB 4EIY) and (b) δOR (PDB 4N6H). The precision of defining the position of individual water molecules (depicted as coloured spheres) is given by the crystallographic b-factors (see colour code). A crystallographic electron density map of water molecules at 1.5σlevel is pictured with COOT software56. 2FO-FCmap is in blue grid and FO-FCmap is in red grid. Figure 1: Water molecules and hydrophobic layers of amino acid residues in the crystal structures of adrenergic and opioid receptors. (a) A 2A R (PDB 4EIY) and (b) δOR (PDB 4N6H). The precision of defining the position of individual water molecules (depicted as coloured spheres) is given by the crystallographic b-factors (see colour code). A crystallographic electron density map of water molecules at 1.5 σ level is pictured with COOT software [56] . 2F O -F C map is in blue grid and F O -F C map is in red grid. Full size image To reveal how water molecules located inside the receptor are distributed spatially and temporally and how they couple to the protein’s structural fluctuations during GPCR activation, we performed all-atom long-timescale MD simulations starting from particular crystal structures of the A 2A R: (a) ZMA antagonist bound to A 2A R (ZMA/A 2A R) representing an inactivated GPCR, (b) agonist NECA docked to inactive A 2A R I (NECA/A 2A R I ) as well as activated A 2A R II crystal structures (NECA/A 2A R II ) representing a GPCR in the meta state between a inactivated and activated receptor, and (c) NECA bound to A 2A R in presence of a C-terminal helix fragment of the G s protein α-subunit (G α ) at the cytoplasmic side (NECA/A 2A R/G α ) representing an activated GPCR/G-protein complex [7] . Two parallel MD simulations of 1.6 μs duration were performed for each of the above-mentioned cases ( Supplementary Table 1 ). Although many water molecules were found inside the receptor during our MD simulations in the case of ZMA/A 2A R, two distinct water-free layers of hydrophobic amino acid side chains were resolved based on water density maps ( Fig. 2a ). These were also revealed from the water molecule distribution in the crystal structure ( Fig. 1a ). The first hydrophobic layer (HL1) was located between the orthosteric and the allosteric sites, and had a thickness of ~7 Å ( Fig. 2a ). Interestingly, water molecules from the bulk next to the bound agonist NECA only rarely diffused into the deep pocket of the receptor. The second hydrophobic layer (HL2) of ~12 Å thickness was located close to the highly conserved NPxxY motif in TM7. In this hydrophobic zone, three interconnected water molecules ( Fig. 1a ) bound to residues between Y288 7.53 and Y197 5.58 in the crystal structure, were broken in the MD simulations and only one water molecule was left connected to Y197 5.58 . This agrees well with the waters’ high mobility indicated by their high b-factors and poor localization in the density maps of the crystal structures. 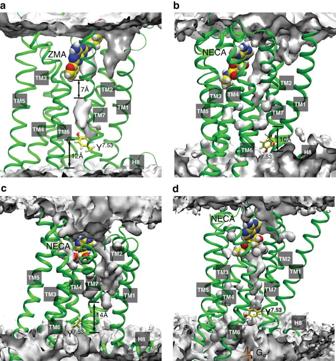Figure 2: Location of the hydrophobic residue layers based on maps of water density inside the A2AR. Final MD structural details of the hydrophobic layer and average water density are shown for (a) ZMA/A2AR, (b) NECA/A2ARI, (c) NECA/A2ARIIand (d) NECA/A2AR/Gα. Figure 2: Location of the hydrophobic residue layers based on maps of water density inside the A 2A R. Final MD structural details of the hydrophobic layer and average water density are shown for ( a ) ZMA/A 2A R, ( b ) NECA/A 2A R I , ( c ) NECA/A 2A R II and ( d ) NECA/A 2A R/G α . Full size image For the activated GPCR in the NECA/A 2A R I complex, many more water molecules were located inside the receptor ( Fig. 2b ) than for the inactive GPCR in the ZMA/A 2A R complex. In ZMA/A 2A R, water molecules from the bulk directly accessed HL1, and in NECA/A 2A R I , the NECA agonist was connected to the NPxxY motif through a network of continuous water molecules involving a sodium ion inside the receptor. In addition, the conformation of Y288 7.53 underwent a single flip-transition during MD simulations in the time range of 0.3–0.6 μs ( Fig. 3c,d ). Superposing the final structure of NECA/A 2A R I from MD simulations (after a residue flip) with the NECA/A 2A R crystal structure [12] , we found that the residue Y288 7.53 adopted identical conformations ( Supplementary Fig. 1a ). Moreover, the HL2 observed in the ZMA/A 2A R complex was retained in the NECA/A 2A R I complex, but the thickness was reduced to ~10 Å ( Fig. 2b ). The HL2 was also observed within two independent additional 1.6 μs MD simulations, starting from the NECA/A 2A R II structure [13] ( Fig. 2c ). 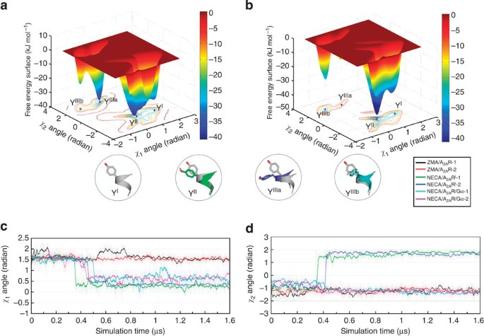Figure 3: Three distinct rotamer states of Y2887.53at the NPxxY motif. (a) Free-energy surface of the agonist NECA bound to A2AR in absence of Gα. (b) Free-energy surface of agonist NECA bound to A2AR in presence of Gαat the cytoplasmic site. (c) Time dependence of angleχ1of Y2887.53during MD simulations of ZMA/A2AR, NECA/A2AR and NECA/A2AR/Gα. (d) Time dependence of angleχ2of Y2887.53for the same complexes. Figure 3: Three distinct rotamer states of Y288 7.53 at the NPxxY motif. ( a ) Free-energy surface of the agonist NECA bound to A 2A R in absence of G α . ( b ) Free-energy surface of agonist NECA bound to A 2A R in presence of G α at the cytoplasmic site. ( c ) Time dependence of angle χ 1 of Y288 7.53 during MD simulations of ZMA/A 2A R, NECA/A 2A R and NECA/A 2A R/G α . ( d ) Time dependence of angle χ 2 of Y288 7.53 for the same complexes. Full size image Notably, during a simulation of the NECA/A 2A R/G α complex with G α present at the cytoplasmic G-protein-binding site, both HLs were no longer detected in the receptor. Instead, a continuous water channel formed spanning from the ligand orthosteric binding site towards the G-protein interaction zone ( Fig. 2d ). Y288 7.53 also performed a flip-rotation transition during the course of MD simulations of NECA/A 2A R/G α ( Figs 2d and 3c,d ), but adopted a conformation distinct from those in crystal structures of ZMA/A 2A R and NECA/A 2A R. Superpositioning the final NECA/A 2A R/G α structure with that of fully activated β 2 AR in complex with G protein (PDB 3SN6) [5] revealed that Y288 7.53 shared the same conformation ( Supplementary Fig. 1b ). HLs in Rho and the β 2 AR To further test our results on HLs in A 2A R, the MD simulations were also performed for two additional receptors, Rho and the β 2A R. As before, 2 × 1.6-μs all-atom MD simulations were performed for three different forms of each receptor. For Rho, we simulated the inactive receptor structure [14] comprising the covalently bound 11- cis- retinal (PDB 1U19; cRET/Rho) as well as the activated receptor structure with bound all- trans -retinal [15] (PDB 2X72) in the presence (tRET/Rho/G α ) and absence of G α (tRET/Rho). Similarly, in the β 2 AR, we investigated the structure of the complex (PDB 2RH1) between the partial inverse agonist carazolol and β 2 AR [16] (CAR/β 2 AR) and between the full agonist BI-167107 and β 2 AR (PDB 3SN6) [17] with G α (BIA/β 2 AR/G α ) and without G α (BIA/β 2 AR) ( Supplementary Table 1 ). Since the HLs changed during MD simulations, we took snapshots from the final 0.3 μs simulations for statisitical analysis. In inactive Rho ( Supplementary Fig. 2a ), we also identified two HLs near the orthosteric site and the NPxxY motif showing a thickness of ~5 Å and ~10 Å, respectively. However, in activated Rho without G α at the cytoplasmic site ( Supplementary Fig. 2b ), HL1 increased to ~7 Å while HL2 disappeared and was replaced by water molecules from the intracellular region. Interestingly, a continuous water channel was found in the structure of the tRET/Rho/G α complex ( Supplementary Fig. 2c ), where both, HL1 and HL2 were accessed by water during MD simulations. Similarly, two layers of hydrophobic amino acid residues were observed in the complex with antagonist CAR/β 2 AR ( Supplementary Fig. 2d ), having a thickness of ~5 Å and ~12 Å, respectively. Different from both A 2A R and Rho, lack of the G α -protein in the activated β 2 AR led to an influx of water molecules from the cytoplasmic side of the receptor, finally forming a continuous water pathway. Furthermore, reorganization of the water molecules also induced Y326 7.53 at the β 2 AR NPxxY motif to flip back to the inactive conformation ( Supplementary Figs 2e and 3 ). These observations agree with the previous findings of Dror et al. [17] that resetting the fully activated β 2A R into the inactivated state requires tenths of a microsecond. The HL as a common feature of GPCRs To further investigate whether the existence of the second layer of hydrophobic residues at the highly conserved NPxxY motif is a common feature of family A GPCRs, we employed a three-dimensional sequence alignment based on all 20 released structures of different members of family A GPCRs. As depicted in Fig. 4 , residues in this second layer were mainly hydrophobic (Val, Leu, Ile, Phe and Pro). Small polar residues (Thr, Ser, Tyr and Met) were a few times also found in this region bound to other hydrophobic residues by their non-polar moieties. There was only one exception, with an Arg in chemokine receptor type 4 (CXCR4) at position 2.43 in transmembrane helix 2 (TM2) [17] . But even in this particular case, the hydrophobic part in the side chain of Arg in the crystal structure was still in a conformation pointing towards the hydrophobic zone, leaving the positively charged moiety directed towards the cytoplasmic region. The recently released 1.8-Å high-resolution DOR crystal structure ( Fig. 1b ) also fits into the above findings [12] . 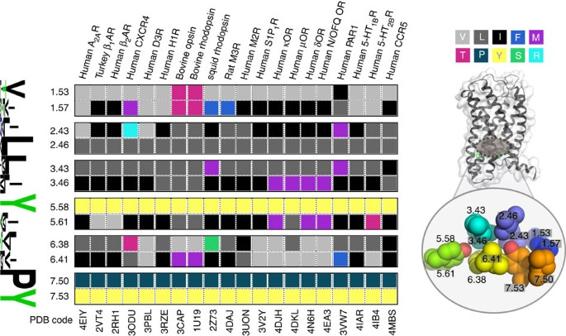Figure 4: The residues comprising the conserved hydrophobic layer located near the NPxxY motif in class A GPCRs. Left: alignment of amino acid residues (depicted in colour code and size according to frequency) in the hydrophobic layer HL2 near the NPxxY motif of 20 class A GPCRs. Right, top: location of HL2 inside a non-activated class A GPCR. Residues are coloured according to their type. Right, bottom: The most conserved residues, P7.50and Y7.53are coloured orange in the image of the GPCR structure. Figure 4: The residues comprising the conserved hydrophobic layer located near the NPxxY motif in class A GPCRs. Left: alignment of amino acid residues (depicted in colour code and size according to frequency) in the hydrophobic layer HL2 near the NPxxY motif of 20 class A GPCRs. Right, top: location of HL2 inside a non-activated class A GPCR. Residues are coloured according to their type. Right, bottom: The most conserved residues, P 7.50 and Y 7.53 are coloured orange in the image of the GPCR structure. Full size image Three different conformations of Y 7.53 From long time scale MD simulations on A 2A R, Rho and β 2 AR, we observed that Y 7.53 , a highly conserved residue in class A GPCRs ( Fig. 4 ), underwent various defined conformational transitions ( Fig. 3 ). In the crystal structures of the analyzed receptors we observed three unique rotamer configurations of Y 7.53 , namely Y I , Y II and Y III ( Fig. 3 ), which correlate with the functional state of GPCRs ( Table 1 ). The Y I conformation is found in many antagonist-bound GPCR structures such as ZMA/A 2A R (ref. 7 ), or in inverted agonist-bound receptors such as CAR/β 2 AR (ref. 16 ). The Y II rotamer is present in agonist-bound receptors, such as BIA/β 2 AR/G α , with G α bound at the cytoplasmic site. The Y III conformation appears in agonist-bound receptors without stabilization by G α such as NECA/A 2A R, or arrestin-biased ligand-bound receptors as in the crystal structure of 5-HT 2B R (ref. 18 ). All three conformations have been distinguished in our simulations, including both classical unbiased long timescale MD simulations as well as in metadynamics simulations (biased). In the classical unbiased MD simulations ( Fig. 3c,d ), starting from the antagonist-bound crystal structure [7] , the residue Y288 7.53 was stabilized at the Y I conformation during the whole 1.6-μs MD simulation of ZMA/A 2A R. However, in the simulations of NECA/A 2A R, a flip-rotation transition to the Y III conformation took place in the 0.3–0.6 μs time range and this rotamer state remained until the end of the simulations. The Y III conformation found in the MD simulations is identical to that in the previously solved crystal structure of A 2A R (PDB 2YDV) [13] . Interestingly, when both the agonist NECA and the Gα protein were present, a transition of Y I to Y II state took place in the 0.3–0.5 μs time range and this rotamer state remained stable until the end of these simulations. Table 1 The Y 7.53 rotamer and the internal water channel structures in relation to the activity states of different ligand/GPCR complexes*. Full size table To investigate the free-energy differences between the different conformations of Y 7.53 we performed a well-tempered metadynamics simulation to estimate free-energy surface (FES). It was done for the agonist NECA-bound A 2A R receptor, in the absence ( Fig. 3a ) and presence ( Fig. 3b ) of G α at its binding site on the receptor. In the metadynanics simulations, two distinct Y III conformations were sampled, Y IIIa and Y IIIb , which differed in the χ 1 angle. In the absence of G α , Y I , Y II and Y IIIa showed similar FES values of −33, −38 and −37 kJ mol −1 , respectively, implying that under these conditions various states can co-exist in the receptor. It is important to note that an alternative Y III conformation Y IIIb , with a FES value of −22 kJ mol −1 , was also sampled. Y IIIb showed a different χ 1 angle with the aromatic ring flipped towards TM1 and TM2. Interestingly, in the presence of G α , the FES for all states, except Y IIIa , decreased by −15 kJ mol −1 , and finally stabilized at values of −34, −47 and −28 kJ mol −1 for Y I , Y II and Y IIIb , respectively. Compared with structures without G α , the FES values indicate that the Y II state is substantially more stable than any other rotamer configuration. Our findings are also supported by the observations of Nygaard et al. [19] that G proteins can stabilize the fully active state of GPCRs, preventing the receptor from switching to different states. These observations tempted us to investigate how the Y 7.53 conformations correlate with a continuous water pathway and the activation of GPCRs. Internal, structured water molecules play a critical role in receptor activation; some of these waters connect two TM helices and some form a H-bond network between receptor and ligand [20] . Closer examination revealed that these water molecules are mobile. The activation of GPCRs is featured by a movement of TM helixes, which opens a large space at the cytoplasmic region for binding a G protein [21] , [22] . Therefore, the activated state of a GPCR can be characterized by the volume change at the G-protein-binding site. According to our simulations, the antagonist-bound complex ZMA/A 2A R ( Fig. 5 ), representing an inactive receptor, shows a relatively small average volume of the G-protein-binding region of VG ~700 Å 3 . In NECA/A 2A R I and NECA/A 2A R, II the A 2A R remains in the meta state [18] , which is between an inactive and active state, showing VG values of ~1,100 Å 3 . It is interesting that in the meta state GPCR crystal structures of NECA/A 2A R and arrestin/5-HT 2B R, the Y 7.53 adopt the Y III conformation [20] , [22] . Moreover, it is known that upon NECA binding the adenosine receptor also signals via arrestin [23] . These findings imply that arrestin-biased activated GPCRs are featured by Y III rotamer. We suggest that our final state of 1.6 μs MD simulation of NECA/A 2A R/G α represents the initial activation stage of A 2A R with a partially activated receptor. 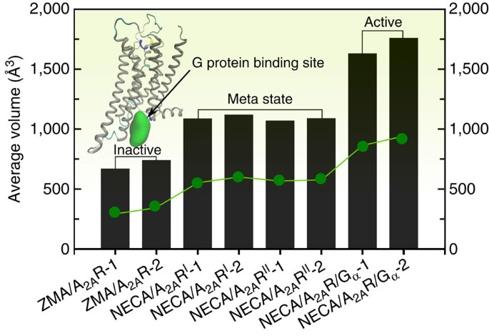Figure 5: Average volume (VG) of the G-protein-binding site in A2AR at different functional states. Non-activated, meta state and activated A2AR are characterized by different volumes. The inactive states show the lowest VG values, the activated receptors have the largest VG values, and VG values of the meta states are between those of inactive and activated GPCR states. For NECA/A 2A R/G α , the receptor’s volume of the binding region for the G protein is VG~1600 Å 3 , which is considerably larger than for ZMA/A 2A R and NECA/A 2A R. Figure 5: Average volume (VG) of the G-protein-binding site in A 2A R at different functional states. Non-activated, meta state and activated A 2A R are characterized by different volumes. The inactive states show the lowest VG values, the activated receptors have the largest VG values, and VG values of the meta states are between those of inactive and activated GPCR states. Full size image In Rho, the VG of the inactive state is also small ( Supplementary Fig. 4 ), adopting a value of ~800 Å 3 . Interestingly, the volumes VG of active tRET/Rho and tRET/Rho/G α are both in the range of ~1,300 Å 3 . The comparison of the VG value in the complex CAR/β 2 AR with the VG values in A 2A R and Rho, show that this volume in a receptor’s inactive state is much smaller than in the active one. Noticeably, the VG of BIA/β 2 AR is comparable with VG of BIA/β 2 AR/G α , although no G α is present at cytoplasmic region in BIA/β 2 AR. This is in agreement with the previous finding [24] that β 2 AR requires tens of microseconds to reset back to inactive states from a fully activated structure. However, we still observed that VG of BIA/β 2 AR already shrunk to ~700 Å 3 compared with fully activated BIA/β 2 AR/G α ( Supplementary Fig. 4 ). G α stabilizes the Y II state of Y 7.53 in various GPCRs To investigate how G protein stabilizes the Y II conformation in the fully activated receptor state, we simulated 2 × 1.6 μs for Rho, β 2 AR and A 2A R, with and without G α ( Fig. 6 ). In the G α -bound receptor state, Y 7.53 was tightly stabilized by residues of the G protein. Specifically, the Y306 7.53 Y II rotamer in Rho ( Fig. 6a ) was bound to R135 3.50 and L349 from the G α protein, Y326 7.53 in Y II state in the β 2A R ( Fig. 6b ) was stabilized by R131 3.50 and Y391 from G α , and the residue Y288 7.53 (Y II ) in the A 2A R ( Fig. 6c ) was stabilized by I292 7.57 and Y391 from G α . Analogously, the Y II state was also seen in two recently published crystal structures of GPCRs with bound agonists, the 5-HT 1B R (ref. 25 ) and the β 2 AR (ref. 16 ) ( Supplementary Fig. 5 ): the Y II conformation in these structures was stabilized by L1048 from the fusion protein and by R147 3.50 , which is present in the G-protein-binding site of 5-HT 1B R. In the β 2A R, the residue I104 from the nanobody Nb80 and residue R131 3.50 stabilized the active Y II state of the receptor. When G α was absent in agonist-bound Rho ( Fig. 6d ), Y306 7.53 was still retained by the hydrophobic moieties of three methionine residues including M257 6.40 , M253 6.36 and M309 7.56 , which have been shown by mutagenesis experiments [26] , [27] to play a role in the activation of Rho. Our MD results are also in agreement with a recently released crystal structure of octylglucoside solubilized Rho without G protein [28] , revealing that the active state of Rho does not need to be stabilized by a G protein. In A 2A R and β 2A R, which are partially activated even in the basal state, the Y II state was not maintained and finally stabilized in Y I ( Fig. 6e ) and Y III ( Fig. 6f ) conformations in complexes with bound agonists and in absence of G α . 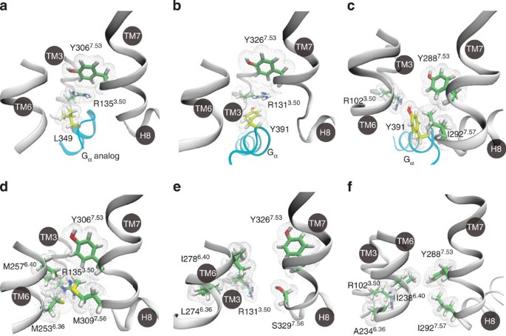Figure 6: Stabilization of of Y7.53in the NPxxY motif. (a) In Rho, Y3067.53is stabilized in the YIIactive state by R1353.50of TM3 and L349 of Gα. (b) In the β2AR, Y3267.53is stabilized in the YIIactive state by R1313.50of TM3 and Y391 of Gα. (c) In the A2AR, Y2887.53is stabilized in the YIIactive state by I2927.57of TM7 and Y391 of Gα. (d) In absence of Gα, Y3067.53is stabilized in the YIIactive configuration by the three Met residues: M2576.40, M2536.36and M3097.56. (e) In absence of Gα, Y3267.53switched back to the inactive YIconfiguration. (f) In absence of Gα, Y2887.53switched to the alternative YIIIconfiguration. Figure 6: Stabilization of of Y 7.53 in the NPxxY motif. ( a ) In Rho, Y306 7.53 is stabilized in the Y II active state by R135 3.50 of TM3 and L349 of G α . ( b ) In the β 2 AR, Y326 7.53 is stabilized in the Y II active state by R131 3.50 of TM3 and Y391 of G α . ( c ) In the A 2A R, Y288 7.53 is stabilized in the Y II active state by I292 7.57 of TM7 and Y391 of G α . ( d ) In absence of G α , Y306 7.53 is stabilized in the Y II active configuration by the three Met residues: M257 6.40 , M253 6.36 and M309 7.56 . ( e ) In absence of G α , Y326 7.53 switched back to the inactive Y I configuration. ( f ) In absence of G α , Y288 7.53 switched to the alternative Y III configuration. Full size image The mechanism of water penetration into GPCRs In our present work we found that GPCRs in their activated state comprise a continuous internal TM water channel. In our previous projects we investigated how water molecules enter the interior of the receptor [8] , [29] . For formyl peptide receptor 1 (FPR 1 ) and opioid receptors (ORs), using microsecond MD simulations, we showed that the influx of water molecules occurs towards the allosteric site, which is different from that in the human sphingosine-1-phosphate receptor 1 (S1PR 1 ) [30] . Jastrzebska et al. [3] reported that water molecules can reach the opsin binding region from the intracellular side during the retinal isomerization in Rho, which is also seen in our MD simulations of Rho. These observations imply that there are two possible water penetration routes. In some receptors, such as Rho and S1PR 1 , the intracellular water penetration occurs when the receptors are being activated, whereas for other receptors, such as ORs and A 2A R, the extracellular water penetration occurs during the activation process. Our analysis of 20 crystal structures of different GPCRs showed that the allosteric ligand binding regions of Rho and S1PR 1 are entirely covered by large N-termini and ECL2 loops (NEL; Fig. 7a , left blue sphere), preventing bulk water molecules from moving towards the central inner space of the receptor. However, for all other receptors, the NELs are much smaller, leaving the orthosteric site widely open ( Fig. 7a , right blue sphere). Closer inspection of the interaction surface area (ISA) between NEL and the remaining moiety of GPCRs ( Fig. 7a ) further confirmed these differences: Rho and S1PR 1 show ISA values of 3,500–4,300 Å 2 , which are much larger than the ISA values of all other receptors ranging between 1,200 and 2,400 Å 2 . Furthermore, the ligand binding layers in Rho and S1PR 1 are more hydrophobic than those in the other GPCRs ( Fig. 7b ). This strong hydrophobic property of Rho and S1PR 1 could further block the water influx from the extracellular bulk environment. Notably, many GPCRs used in X-ray crystallography were strongly modified to allow crystallization, for example, sometimes the flexible N-termini were cut or additional protein sequences were inserted into certain receptor loops. Nevertheless, it is still acceptable to compare the ISA contact areas in the crystal structures, since the flexible modified regions may not contribute much to the contact area as they might be disordered under physiological conditions. 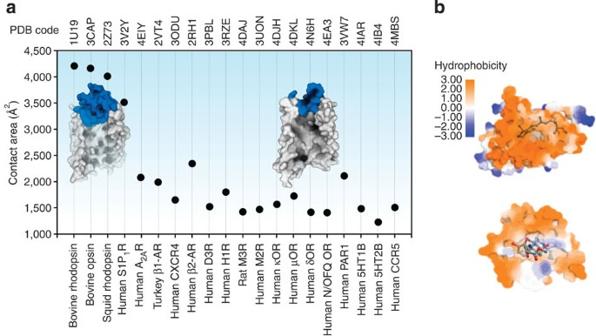Figure 7: Contact areas between EL2 and the N-terminus in GPCRs. (a) Inspection of crystal structures of 20 different GPCRs show two receptor clusters: Receptors similar to Rho and S1PR1have a high contact area of 3,500–4,300 Å2. The remaining receptors have a low contact area of 1,200–2,400 Å2. (b) Hydrophobicity profile of the ligand binding site in rhodopsin (top) and in the μ-OR (bottom); colours: orange, hydrophobic surface; blue, polar surface. Figure 7: Contact areas between EL2 and the N-terminus in GPCRs. ( a ) Inspection of crystal structures of 20 different GPCRs show two receptor clusters: Receptors similar to Rho and S1PR 1 have a high contact area of 3,500–4,300 Å 2 . The remaining receptors have a low contact area of 1,200–2,400 Å 2 . ( b ) Hydrophobicity profile of the ligand binding site in rhodopsin (top) and in the μ-OR (bottom); colours: orange, hydrophobic surface; blue, polar surface. Full size image More than 800 human GPCRs allow cells to recognize diverse extracellular stimuli and transduce signals across the plasma membrane to regulate central physiological processes. Currently, >20 GPCR crystal structures have been solved, but details of their activation are still not fully understood. On the basis of a total of 32-μs all-atom MD simulations, we here analyzed the activation of three different receptors of class A GPCRs. We discovered a specific common feature of the receptors—an intrinsic water pathway, which in the receptors’ resting state is interrupted by a HL of amino acid residues and upon agonist binding, opened to a continuous intrinsic water channel ( Fig. 8 ). Water from the bulk can enter into the receptor during activation from two different directions: from the extracellular ( Fig. 8a ) and from the intracellular side ( Fig. 8b ) depending on the receptor type. Three distinct rotamer conformations, namely Y I , Y II and Y III , of a highly conserved Tyr (Y 7.53 ) residue in the NPxxY motif correlate with the formation of the internal water pathway and the functional state of GPCRs. The Y I state represents the inactive state of receptor with the first layer of hydrophobic amino acid residues located close to the NPxxY motif, the second layer of hydrophobic amino acids next to Y 7.53 and a water pathway is interrupted ( Fig. 8c ). The Y II state indicates fully activated GPCR state with a G protein bound and a continuous water pathway connecting Y 7.53 to extracellular or intracellular side ( Fig. 8a,b ). The Y III state corresponds to the meta state of the receptor comprising a HL next to Y 7.53 ( Fig. 8d ). These findings contribute to better understanding of a role of internal waters in the activation process of GPCRs and provide important new directions for MD-based design of compounds targeting GPCRs. 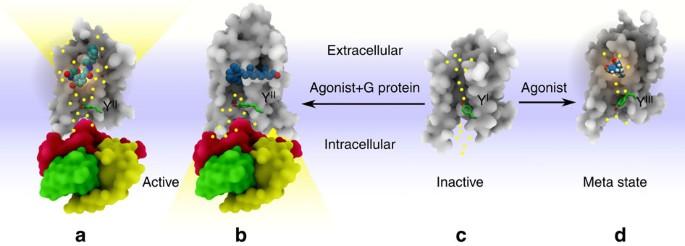Figure 8: A schematic view of three different rotamer conformations of the highly conserved Y7.53residue. (a) The YIIconformation is preferred in activated GPCRs; during formation it is accessed by extracellular water molecules forming a continuous internal water network. (b) For receptors similar to Rho and S1PR1the YIIstate is associated with the cytoplasmic influx of water. GPCRs are shown in grey and the G-protein subunits are displayed in different colours. (c) The YIconformation is preferred in inactive GPCRs with two hydrophobic layers blocking a continuous water pathway. (d) The YIIIconformation is preferred in GPCR meta states with one hydrophobic layer located next to the NPxxY motif and blocking formation of a continuous water pathway. Figure 8: A schematic view of three different rotamer conformations of the highly conserved Y 7.53 residue. ( a ) The Y II conformation is preferred in activated GPCRs; during formation it is accessed by extracellular water molecules forming a continuous internal water network. ( b ) For receptors similar to Rho and S1PR 1 the Y II state is associated with the cytoplasmic influx of water. GPCRs are shown in grey and the G-protein subunits are displayed in different colours. ( c ) The Y I conformation is preferred in inactive GPCRs with two hydrophobic layers blocking a continuous water pathway. ( d ) The Y III conformation is preferred in GPCR meta states with one hydrophobic layer located next to the NPxxY motif and blocking formation of a continuous water pathway. Full size image Loop filling and refinements Since the intracellular loop ICL2 for each receptor was missing because of the insertion of a fusion protein in this region, the loop refinement protocol in Modeller V9.10 was used to fulfil and refine this area [31] . A total of 20,000 loops were generated for each receptor and a conformation with the lowest Discrete Optimized Protein Energy (DOPE) score was chosen for receptor construction. Repaired models were submitted to Rosetta V3.4 for loop refinement with kinematic loop modelling methods [32] . Kinematic closure (KIC) is an analytic calculation inspired by robotics techniques for rapidly determining the possible conformations of linked objects subject to constraints. In the Rosetta KIC implementation, 2N-6 backbone torsions of an N-residue peptide segment (called non-pivot torsions) are set to values drawn randomly from the Ramachandran space of each residue type, and the remaining six φ/ψ torsions (called pivot torsions) are solved analytically by KIC. Protein structure preparations All protein models were prepared in Schrodinger suite software under OPLS_2005 force field. Hydrogen atoms were added to repaired crystal structures at physiological pH (7.0) with the PROPKA (ref. 33 ) tool in Protein Preparation tool in Maestro [33] , [34] , [35] to optimize the hydrogen bond network. Constrained energy minimizations were conducted on the full-atomic models, with heavy atom coverage to 0.4 Å. Models of the receptor/G α complexes were prepared as previously reported [21] . Ligand structure preparations All ligand structures were obtained from the PubChem [36] online database. The LigPrep module in Schrodinger 2012 suite software was introduced for geometric optimization by using OPLS_2005 force field. Ionization states of ligands were calculated with the Epik tool [37] employing Hammett and Taft methods in conjunction with ionization and tautomerization tools. Protein-ligand docking The docking procedure was performed by Glide [38] , [39] . Ligand molecules were initially placed in the binding pocket in a pose similar to that noted in the ligand-bound crystal structure. Cubic boxes centered on the ligand mass centre with a radius 8 Å for all ligands defined the docking binding regions. Flexible ligand docking was executed for all structures. Twenty poses per ligand out of 20,000 were included in the post-docking energy minimization. The best scored pose for each ligand was chosen as the initial structure for MD simulations. MD simulations The membrane system was built by the g_membed [40] tool in Gromacs [41] V4.6.3 with the receptor crystal structure pre-aligned in the Orientations of Proteins in Membranes (OPM) database [42] , [43] . Pre-equilibrated 132 POPC lipids coupled with 9,200 TIP3P water molecules in a box ~70 Å × 70 Å × 98 Å were used for building the protein/membrane system. We modelled the protein using Amber99SB-ILD* force field [44] with improved side-chain torsion potentials of Amber99SB force field. For the POPC lipids, we used the Amber Slipids (Stockholm lipids) force field parameter set, which in recent MD simulations of lipid bilayers yielded excellent agreement with experimental data (X-ray and neutron diffraction; NMR order parameters) [45] , [46] . For modelling the ligand we used the Amber GAFF small molecule force field [47] . The parameters of covalently bound 11- cis -retinal were obtained from a previous report [48] . The ligand geometry was submitted to the GAUSSIAN 09 programme [49] for optimization at Hartree-Fock 6-31G* level, when generating force filed parameters. The system was gradually heated from 0 to 310 K followed by 1 ns initial equilibration at constant volume and temperature set at 310 K. Next, an additional 40 ns constrained equilibration was performed at constant pressure and temperature (NPT ensemble; 310 K, 1 bar), and the force constant was trapped off gradually from 10 to 0 kcal mol −1 . All bond lengths to hydrogen atoms were constrained with M-SHAKE. Van der Waals and short-range electrostatic interactions were cut off at 10 Å. Long-range electrostatic interactions were computed by the Particle Mesh Ewald summation scheme. MD simulations results were analyzed in Gromacs [41] and VMD [50] . Average water density calculation Water density was calculated in Volmap plugin in VMD [50] . Volmap creates a map of the weighted atomic density at each gridpoint. This is done by replacing each atom in the selection with a normalized Gaussian distribution of width (standard deviation) equal to its atomic radius. The Gaussian distribution for each atom is then weighted using an optional weight read from one of the atoms’ numerical properties, and defaults to a weight of one. The various Gaussians are then additively distributed on a grid. The meaning of final map will depend of the weight of mass. The average water density was calculated based on the final 0.3-μs frame of each long time scale MD simulation. Final output results were visualized in VMD. Contact map calculation The contact map for residues at G-protein-binding site was done by g_mdmat in Gromacs that makes distance matrices consisting of the smallest distances between residue pairs. Frames (0.3 μs) of each long time scale MD simulation was used for contact map calculations. Metadynamics simulations Free-energy profiles of the systems were calculated by using well-tempered metadynamics in Gromacs V4.6.3 (ref. 41 ) with Plumed V1.3 patches (ref. 51 ). Metadynamics adds a history-dependent potential V(s, t) to accelerate sampling of the specific collective variables (CVs) s (s 1 , s 2 , …, s m ) [52] . V(s, t) is usually constructed as the sum of multiple Gaussians centred along the trajectory of the CVs (equation 1). Periodically during the simulation, another Gaussian potential, whose location is dictated by the current values of the CVs, is added to V(s, t) (ref. 21 ). In our simulations, the dihedral angles of Y288 7.53 , χ 1 and χ 2 , were assigned as the CVs s 1 and s 2 , while the width of Gaussians, σ , was set as 5 degrees. The time interval τ was 0.09 ps. Well-tempered metadynamics involves adjusting the height, w j , in a manner that depended on V(s, t) , where the initial height of Gaussians w was 0.03 kcal mol −1 , the simulation temperature was 310 K and the sampling temperature Δ T was 298 K. The convergence of our simulations was judged by using the free-energy difference between states X and A at 10-ns intervals. Once the results stopped changing over time, the simulation was considered as converged [53] . Each metadynamics simulation lasted for 140 ns, and the results were analyzed upon convergence. Reweighting algorithm From a converged metadynamics run we can calculate directly the canonical probability distribution of the CVs at a given temperature. On the contrary, the statistics of other degrees of freedom is somehow distorted by the application, during the simulation, of a time-dependent external potential on the CVs. In well-tempered metadynamics, the reconstruction of the distribution of variables different from the CVs is particularly simple since for long time periods the amount of bias added decreases to zero and the system approaches equilibrium. The algorithm described by Bonomi et al. [54] consists of three different steps: (1) Accumulate the histogram of the CVs plus the other variables of interest between two updates of the bias potential. (2) When a new Gaussian is added, evolve the histogram as equation (2): where P ( R , t ) is the biased probability distribution, V ( S ( R ), t ) the time derivative of the bias potential and the average in the exponent is calculated in biased ensemble. (3) At the end of the simulation, the unbiased distribution P B ( R ) can be recovered from the histogram collected by using a standard umbrella sampling reweighting as equation (3): Contact area and binding volume calculations Contact areas between the ECL2/N-terminal and the left space of receptors were calculated by the contact_surface module in Pymol. It calculates individual or global contact areas between a receptor molecule and a (multimodel) bundle of ligand partner structures. The exact contact surface area values are in Å 2 . If only a single global contact surface is calculated, a selection named ‘contact’ is created that includes all receptor atoms within 3.9 Å of any ligand atom to illustrate the approximate contact surface. The average G-protein-binding volumes at the cytoplasmic region were carried out in POVME (ref. 55 ). After filling the defined box with grid points at a 2-Å resolution, the grid points that overlapped with any atom based on van der Waals clashes were removed by ContiguousSeedSphere and ContiguousSeedBox in POVME. A spherical region positioned at the box centre with a 5-Å radius was defined as the core region. Only points that were contiguous with points in the core region were considered. Then the volume was calculated as the summation of the volumes occupied by each remaining point. How to cite this article : Yuan, S. et al. Activation of G-protein-coupled receptors correlates with the formation of a continuous internal water pathway. Nat. Commun . 5:4733 doi: 10.1038/5733 (2014).